A mechanically sensitive cell layer regulates the physical properties of theArabidopsisseed coat Endogenous mechanical stresses regulate plant growth and development. Tensile stress in epidermal cells affects microtubule reorientation and anisotropic cell wall deposition, and mechanical stimulus at the meristem regulates trafficking and polar localization of auxin transporters. However, the mechanical regulation of other plant growth regulators has not been demonstrated. Here we propose that during seed growth, mechanical stress exerted by the expanding embryo and endosperm is perceived by a specific mechanosensitive cell layer in the seed coat. We show that the adaxial epidermis of the outer integument thickens its cell wall in a mechanosensitive fashion, demonstrates microtubule dynamics consistent with mechanical stress perception and shows mechanosensitive expression of ELA1 , a regulator of seed size and gibberellic acid (GA) metabolism. By exploiting physical and genetic compartmentalization, and combining genetic and surgical techniques, we propose a mechanistic link between mechanical stress and GA accumulation that regulates seed development. Studies of mechanical signalling in plant tissues at the cellular level are hampered by the difficulty of distinguishing responses to mechanical signals from those related to wounding and/or changes in intercellular communication. The Arabidopsis seed is comprised of the embryo, endosperm and seed coat, each of which is genetically distinct. Its small size and relative accessibility, and the availability of high quality in silico transcriptome resources [1] , make it an attractive model system. Histological and genetic studies suggest that no symplastic connections exist between the seed coat and the endosperm [2] , [3] . The possibility that mechanical signalling could be involved in coordinating seed development has been evoked previously by studies showing that final seed size is determined by the interplay of expansion of the syncytial endosperm soon after fertilization (controlled by a pathway involving the receptor kinase HAIKU2 (IKU2)) with the regulated growth of the surrounding seed coat [4] . In plants, growth is thought to be restricted by the epidermal cell layer and driven by the combined turgor pressure of cells underlying this cell layer. This generates tissue tension in the epidermis, which is counteracted by thickening of the outer epidermal cell wall [5] , [6] , [7] . At fertilization, the Arabidopsis seed coat is composed of four to five living cell layers derived from two organs, the outer integument (two cell layers; abaxial (outer) epidermis (oi-ab) and adaxial (inner) epidermis (oi-ad)) and the inner integument (abaxial epidermis (ii-ab) and adaxial epidermis (endothelium), separated by one internal cell layer in more chalazal zones of the seed coat) ( Fig. 1a ). The outer cell layer of the developing Arabidopsis seed (oi-ab) differentiates into a highly specialized cell type designed for rupture and release of mucilage on seed imbibition [8] , [9] . In contrast, the cell wall separating oi-ad from ii-ab (‘wall 3’) has been described as being thickened, based upon histological observations [8] , [9] , suggesting that it could restrict seed growth. 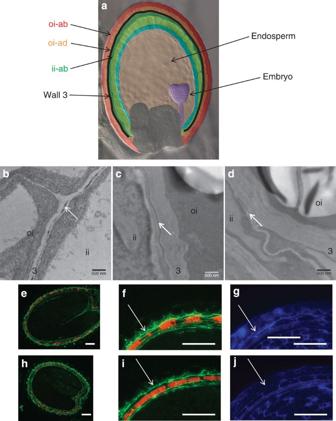Figure 1: The adaxial epidermis of the outer integument is the origin of the thickest cell wall in the seed and shows reduced thickening iniku2-2mutant seed. (a) Developing seed. The seed coat surrounds the endosperm. Wall 3 (3) is situated between oi-ad and ii-ab. (b–d) Transmission electron micrographs of wall 3. (b) Young seed (globular embryo four-cell stage), (c) seed with expanding embryo (walking-stick stage). (d) Seed with fully expanded embryo. White arrows indicate the fusion zone within wall three. Scale bars, 500 nm. (e–j) Comparison of wall 3 immunohistochemical properties in 15 DAP wild-type andiku2-2mutant seed. Seed from wild-type (e–g) andiku2-2mutant (h–j) subjected to immunolocalization with LM19 rat monoclonal antibody (green ine,f,h,i) and then post-stained with calcofluor white (blue ing,j). Red colouration is autofluorescence from the endothelium (ii-ad). Wall 3 is indicated with an arrow in (f,g,i,j). Scale bar, 100 μm ine,hand 50 μm inf,g,i,j. Figure 1: The adaxial epidermis of the outer integument is the origin of the thickest cell wall in the seed and shows reduced thickening in iku2-2 mutant seed. ( a ) Developing seed. The seed coat surrounds the endosperm. Wall 3 (3) is situated between oi-ad and ii-ab. ( b – d ) Transmission electron micrographs of wall 3. ( b ) Young seed (globular embryo four-cell stage), ( c ) seed with expanding embryo (walking-stick stage). ( d ) Seed with fully expanded embryo. White arrows indicate the fusion zone within wall three. Scale bars, 500 nm. ( e – j ) Comparison of wall 3 immunohistochemical properties in 15 DAP wild-type and iku2-2 mutant seed. Seed from wild-type ( e – g ) and iku2-2 mutant ( h – j ) subjected to immunolocalization with LM19 rat monoclonal antibody (green in e , f , h , i ) and then post-stained with calcofluor white (blue in g , j ). Red colouration is autofluorescence from the endothelium (ii-ad). Wall 3 is indicated with an arrow in ( f , g , i , j ). Scale bar, 100 μm in e , h and 50 μm in f , g , i , j . Full size image Here we show not only that wall 3 is thickened in a mechanosensitive manner specifically by oi-ad, but that this cell layer also shows microtubule dynamics consistent with mechanical stress perception and the mechanosensitive expression of a regulator of seed size and gibberellic acid (GA) metabolism. To determine from which cell layer the material in wall 3 originates, we observed developing seeds by transmission electron microscopy. In seeds containing expanding and fully expanded embryos, wall 3 is the thickest periclinal cell wall in the seed coat ( Supplementary Fig. 1 and Fig. 1 ). Consistent with it representing a zone of fusion between two epidermal surfaces, an electron-dense layer of cutin-like material is observed within wall 3 at early stages of seed development ( Fig. 1b ), and remains visible throughout much of the seed development, ‘marking’ the original boundary between the two integuments. Observation of the asymmetric positioning of this zone at later developmental stages shows that the vast majority of cell wall material laid down in wall 3 originates from oi-ad ( Fig. 1c,d ). Because epidermal cells are known to thicken their cell walls in response to mechanical stress [5] , [6] , [7] , we hypothesized that oi-ad might be the site of response to physical stretching imposed by early endosperm expansion. We, therefore, compared the histological and immunohistological observations of wall 3 in wild-type seeds 15 DAP, with haiku2 ( iku2-2 (ref. 10 )) mutant seeds in which early endosperm expansion is dramatically reduced. In the latter, wall 3 stains less strongly with calcofluor (staining cellulose), and with the monoclonal antibody LM19 (which detects de-esterified homogalacturonan [11] ), suggesting that it is thinner in iku2 mutants ( Fig. 1e–j ). Since IKU2 is expressed in the endosperm [10] , we propose that thickening is controlled non-autonomously by endosperm expansion. Microtubule orientation and bundling change in the presence of mechanical stresses in growing tissues and can therefore be used as a marker of stress patterns [12] , [13] , [14] , [15] , [16] . We documented microtubule behaviour in the cells of oi-ab and oi-ad before and after fertilization using lines expressing a GFP (green fluorescent protein) fusion to Tubulin Alpha 6 (ref. 17 ) or an red fluorescent protein fusion to MAP65 (ref. 18 ), which mark microtubules and bundled microtubules, respectively. Microtubules within the oi-ab of unfertilized ovules are arranged in arrays along the short axis of the cell ( Supplementary Fig. 2 and Fig. 2a,b ). Post fertilization, microtubules reorganize and become randomly orientated within each cell, with no evident bundling or supracellular organization observed ( Fig. 2e,f ). After 72–96 h, microtubules start to coalesce at a point in the centre of each cell corresponding to the position of the future columella ( Supplementary Fig. 3 ). In contrast, microtubules in oi-ad become increasingly highly bundled post fertilization ( Fig. 2g,h ) in comparison with non-fertilized controls ( Fig. 2c,d ), with supracellular organization visible. Differences in bundling between the outer and inner cell layer are particularly dramatic when MAP65 is observed ( Fig. 2f compared to Fig. 2h ). The images shown in Fig. 2 are typical of the situation observed in three independent time courses and in at least 10 individual seeds for every time point. To confirm that the microtubules of oi-ab are capable of reorienting in response to mechanical stress, we developed a technique for compressing developing seeds within siliques, whilst still attached to the mother plant ( Supplementary Fig. 4 ). Dissecting and imaging seeds expressing the Lti6b marker [19] after long (24 h) compressions in this apparatus confirms that seed coats are distorted, but not damaged ( Supplementary Fig. 5 ). After 24 h of compression in this apparatus, we found that microtubules in oi-ab had undergone a dramatic reorientation, suggesting that they are capable of responding to mechanical stresses, but are not subject to such stresses during normal development ( Fig. 2i–k ). Although we are unable to visualize microtubules in deeper cell layers for technical reasons, these observations, together with the presence of cell wall thickening, support the hypothesis that oi-ad is the major site for the perception of, and response to, mechanical stresses during normal seed development. 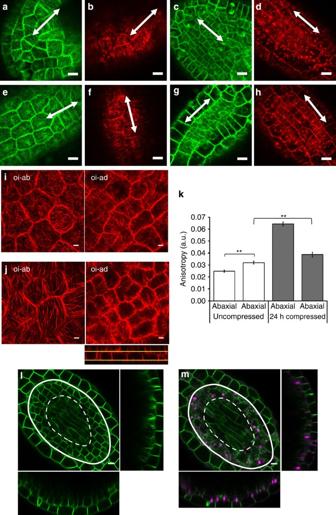Figure 2: Microtubule dynamics in the adaxial epidermis of the outer integument are consistent with the perception of mechanical tension in this cell layer post fertilization. Control unfertilized ovules (a–d) and seeds at 72 h after pollination (e,f) expressing TUA6-GFP (a,c,e,g) or MAP65-RFP (b,d,f,h).a,b,e,fandc,d,g,hfocus on oi-ab and oi-ad, respectively. The long axis of the ovule/seed is indicated by a double-headed arrow. (i–k) Microtubules in oi-ab can bundle and reorient in response to mechanical stress. MAP65-RFP-expressing seeds 48 h after fertilization were either compressed (j) or left uncompressed (i) for 24 h before imaging of microtubule arrays in oi-ad and oi-ab. Positions of sections are indicated by yellow lines in orthogonal projection inj. (k) Microtubule anisotropy was measured for both cell layers in control and compressed seeds. A significant difference in anisotropy is observed between oi-ab and oi-ad in controls. Compression leads to more markedly increased anisotropy in oi-ab, suggesting that this cell layer is not under significant mechanical tension in uncompressed seeds, but can respond strongly to applied tension. Results were generated in two independent experiments using cells from at least 10 seeds for each condition.N(number of cells analysed)=304 and 176 respectively for oi-ab and oi-ad in uncompressed conditions, and 311 and 88, respectively, for oi-ab and oi-ad in compressed conditions. **P<0.01, Student’st-test. (l) Optical section of seed coat before endosperm blow-out surgery showing intact oi-ab (outer area), oi-ad (between solid and hashed rings) and ii-ab (inside hashed ring). (m) The same seed post surgery (puncture site below plane of focus). Propidium iodide staining is shown in magenta. Further sections are shown inSupplementary Fig. 7. Scale bar, 10 μm. Figure 2: Microtubule dynamics in the adaxial epidermis of the outer integument are consistent with the perception of mechanical tension in this cell layer post fertilization. Control unfertilized ovules ( a – d ) and seeds at 72 h after pollination ( e , f ) expressing TUA6-GFP ( a , c , e , g ) or MAP65-RFP ( b , d , f , h ). a , b , e , f and c , d , g , h focus on oi-ab and oi-ad, respectively. The long axis of the ovule/seed is indicated by a double-headed arrow. ( i – k ) Microtubules in oi-ab can bundle and reorient in response to mechanical stress. MAP65-RFP-expressing seeds 48 h after fertilization were either compressed ( j ) or left uncompressed ( i ) for 24 h before imaging of microtubule arrays in oi-ad and oi-ab. Positions of sections are indicated by yellow lines in orthogonal projection in j . ( k ) Microtubule anisotropy was measured for both cell layers in control and compressed seeds. A significant difference in anisotropy is observed between oi-ab and oi-ad in controls. Compression leads to more markedly increased anisotropy in oi-ab, suggesting that this cell layer is not under significant mechanical tension in uncompressed seeds, but can respond strongly to applied tension. Results were generated in two independent experiments using cells from at least 10 seeds for each condition. N (number of cells analysed)=304 and 176 respectively for oi-ab and oi-ad in uncompressed conditions, and 311 and 88, respectively, for oi-ab and oi-ad in compressed conditions. ** P <0.01, Student’s t -test. ( l ) Optical section of seed coat before endosperm blow-out surgery showing intact oi-ab (outer area), oi-ad (between solid and hashed rings) and ii-ab (inside hashed ring). ( m ) The same seed post surgery (puncture site below plane of focus). Propidium iodide staining is shown in magenta. Further sections are shown in Supplementary Fig. 7 . Scale bar, 10 μm. Full size image To test this hypothesis further, we surgically altered the turgor pressure applied by the expanding syncytial endosperm on the seed coat. We imaged developing seeds expressing the membrane marker Lti6b-GFP, 6 days after fertilization (early heart stage, endosperm uncellularized ( Supplementary Fig. 6 for staging)). We then gently ‘blew out’ the endosperm by microinjecting a small bubble of air into the endosperm cavity and reimaged the seeds within 15–20 min. Pre-surgery imaging allows clear visualization of the membranes of oi-ab, oi-ad and the underlying ii-ad (composed of characteristic elongated cells; Fig. 2l,m and Supplementary Fig. 7 ). Membranes lose their integrity in oi-ad post surgery, despite the fact that those in over- and underlying cell layers can still be clearly observed (100% n =30 seeds). When post-surgery seeds are imaged in the presence of propidium iodide (which does not enter intact seeds at this stage), we observe strong uniform nuclear staining specifically in oi-ad, suggesting that these cells lose their integrity in response to the changes in mechanical stress imposed on them ( Fig. 2l,m and Supplementary Fig. 7 ). Oi-ad thus appears to be particularly sensitive to mechanical perturbation. After endosperm cellularization initiates at the early heart stage in wild-type seeds, seed size does not increase significantly. However, in plants heterozygous for a recessive loss of function mutation in the ZHOUPI (ZOU) gene, which encodes an endosperm-specific bHLH transcription factor necessary for endosperm breakdown as the embryo starts to expand at the early torpedo stage [20] , [21] , [22] , we find that seeds containing a mutant endosperm and embryo become significantly larger than their siblings before desiccation ( Supplementary Fig. 8 ). We hypothesized that this could be due to competition for space within the seed coat, between the persistent endosperm and the expanding embryo. We interrogated available transcriptional data generated in zou-4 mutant versus wild-type seeds at the mid torpedo stage of embryo development [22] to identify genes expressed in the seed coat (based on in silico data [1] ) and upregulated in the zou-4 mutant background. One such gene is At5g24910 , which encodes the cytochrome p450 mono-oxygenase CYP714A1, also named EUI-LIKE P450 A1 (ELA1) [23] , [24] . Upregulation of ELA1 in zou mutants is confirmed using quantitative reverse transcription PCR ( Fig. 3a ). ELA1 is also significantly upregulated in iku2 mutants at the torpedo stage, and more strongly upregulated in zou-4 iku2-2 double mutants than in either single mutant. In zou-4 iku2-2 double mutants we note a significantly decreased seed viability, due to testa rupture in 30–50% of developing seeds ( Supplementary Fig. 9 ). We propose that the lack of wall 3 strengthening in iku2 mutants leads to increased oi-ad stretching during embryo growth, and that this is compounded by endosperm persistance in zou-4 iku2-2 double mutants, leading to testa rupture ( Fig. 4e ). 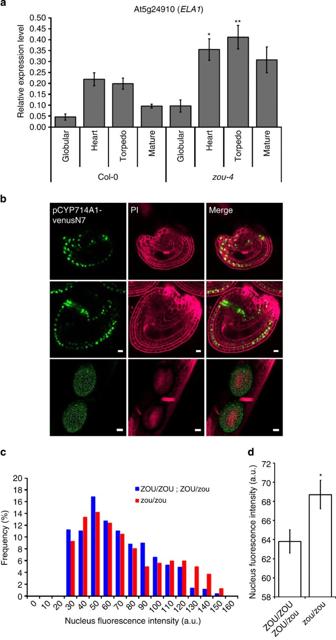Figure 3: Expression ofELA1is upregulated inzou-4mutants and largely restricted to the adaxial cell layer of the outer integument. (a) Quantitative reverse transcription PCR analysis ofELA1expression relative to that ofEIF4Ain wild-type andzou-4mutant siliques. Error bars are s.e. from at least three biological replicates. *P<0.05 and **P<0.01, Student’st-test. (b) Confocal images of a propidium iodide (magenta) stained ovule (top row) and young seeds (second and third rows) expressing thepELA1:VENUS-N7construct (green). First and second rows are optical sections, whilst row three is a reconstituted stack. Scale bars, 10 μm in the top two rows and 100 μm in the bottom row. (c) Nucleus fluorescence quantification in seeds ofpELA1:VENUS-N7plants heterozygous forzou-4.Nucleus fluorescence was measured in multiple seeds from four siliques (ZOU/ZOU+ZOU/zouN= 535,zou/zou N=486). (d) Average fluorescence fromc, *P<0.05, Student’st-test. Figure 3: Expression of ELA1 is upregulated in zou-4 mutants and largely restricted to the adaxial cell layer of the outer integument. ( a ) Quantitative reverse transcription PCR analysis of ELA1 expression relative to that of EIF4A in wild-type and zou-4 mutant siliques. Error bars are s.e. from at least three biological replicates. * P <0.05 and ** P <0.01, Student’s t -test. ( b ) Confocal images of a propidium iodide (magenta) stained ovule (top row) and young seeds (second and third rows) expressing the pELA1:VENUS-N7 construct (green). First and second rows are optical sections, whilst row three is a reconstituted stack. Scale bars, 10 μm in the top two rows and 100 μm in the bottom row. ( c ) Nucleus fluorescence quantification in seeds of pELA1:VENUS-N7 plants heterozygous for zou-4. Nucleus fluorescence was measured in multiple seeds from four siliques ( ZOU/ZOU+ZOU/zou N= 535, zou/zou N =486). ( d ) Average fluorescence from c , * P <0.05, Student’s t -test. 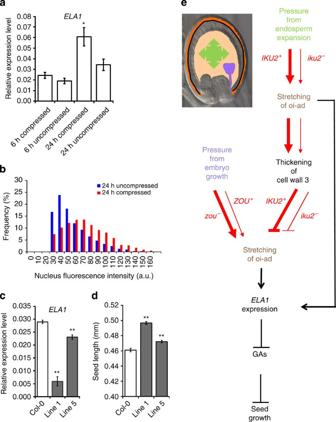Figure 4: TheELA1gene shows mechanoresponsive expression and is involved in regulating seed coat mechanical properties. Quantitative reverse transcription PCR (qPCR) analysis ofELA1expression relative to the expression ofEIF4Ain 6 dap siliques compressed using apparatus described inSupplementary Fig. 4. Error bars are s.e. from eight biological replicates. (b) Nucleus fluorescence quantification from identical experiments carried out on plants expressing thepELA1:VENUS-N7construction (seeSupplementary Fig. 11for images and data at 6 h).N=992 in control and 1,020 in compressed samples at 24 h. Similar results were obtained in two independent experiments. (c) qPCR analysis ofELA1expression levels in two independent amiRNA knockdown lines (for details, seeSupplementary Fig. 14). Error bars are s.e. from six biological replicates. (d) Seed length measurements from lines are shown inc. Col0N=140, line 1N=280, line 5N=280. *P<0.05, **P<0.01, Student’st-test. (e) Proposed model relating responses to mechanical stresses perceived in oi-ab with GA-mediated seed growth control. Full size image Figure 4: The ELA1 gene shows mechanoresponsive expression and is involved in regulating seed coat mechanical properties. Quantitative reverse transcription PCR (qPCR) analysis of ELA1 expression relative to the expression of EIF4A in 6 dap siliques compressed using apparatus described in Supplementary Fig. 4 . Error bars are s.e. from eight biological replicates. ( b ) Nucleus fluorescence quantification from identical experiments carried out on plants expressing the pELA1:VENUS-N7 construction (see Supplementary Fig. 11 for images and data at 6 h). N =992 in control and 1,020 in compressed samples at 24 h. Similar results were obtained in two independent experiments. ( c ) qPCR analysis of ELA1 expression levels in two independent amiRNA knockdown lines (for details, see Supplementary Fig. 14 ). Error bars are s.e. from six biological replicates. ( d ) Seed length measurements from lines are shown in c . Col0 N =140, line 1 N =280, line 5 N =280. * P <0.05, ** P <0.01, Student’s t -test. ( e ) Proposed model relating responses to mechanical stresses perceived in oi-ab with GA-mediated seed growth control. Full size image The seed expression pattern of ELA1 was investigated by both in situ hybridization ( Supplementary Fig. 10 ) and by the generation of a promoter fusion to a sequence encoding the nuclear VENUS-N7 protein fusion ( Fig. 3b ). ELA1 is expressed most strongly in oi-ad, with weaker expression also observed in the internal cell layer of the inner integument at early stages. Using the apparatus described previously ( Supplementary Fig. 4 ), we observe that the transcript levels of ELA1 respond positively to the application of exogenous mechanical stress after 24 h of compression ( Fig. 4a ). When identical experiments are carried out on lines expressing pELA1:VENUS-N7 , no ectopic expression of this marker is observed ( Supplementary Fig. 11a ), suggesting that increased transcript levels are restricted to the native expression domain. Quantification of nuclear fluorescence in these lines supports an upregulation in the activity of the ELA1 promoter both following seed compression ( Fig. 4b and Supplementary Fig. 11b ) and in seeds containing zou-4 mutant endosperm and embryo ( Fig. 3c,d ). In contrast, the expression of RGP4 (ref. 25 ) and At1g63300 , two other seed coat-specific genes showing similar global expression profiles to ELA1 , ELA2 , a close homologue and direct physical neighbour of ELA1 (ref. 23 ) and RGP3 , an endosperm-specific gene [25] , is not affected by mechanical stress application ( Supplementary Fig. 12 ). Although the loss of ELA1 function alone does not affect the seed size, ELA1 , together with ELA2 , has previously been shown to restrict seed expansion [23] . However, ELA2 is expressed both in the seed coat and in the endosperm ( Supplementary Fig. 13 ). We therefore generated amiRNA lines targeting both ELA1 and ELA2 under the ELA1 promoter ( Supplementary Fig. 14a,b ). Although the plants are otherwise phenotypically normal, we detect statistically significant increases in seed length and area in two independent lines showing reduction in ELA1 expression ( Fig. 4c,d and Supplementary Fig. 14c ), confirming that ELA1 and ELA2 act together in the seed coat to limit seed size. The control of final seed size in angiosperms is known to involve a fine balance between endosperm expansion and controlled seed coat extension. We interpret our observations of cytoskeletal behaviour, micromanipulations and structural studies in wild-type and iku2 mutants as suggesting that the control of seed coat extension involves mechanoresponsive cell wall thickening by the adaxial epidermis of the outer integument. On the basis of our results, we propose that early in seed development this layer senses mechanical stresses exerted on the seed coat by the expanding syncytial endosperm and reacts by reinforcing its ‘outer’ cell wall (wall 3) to form a ‘corset’ around the developing seed. Our analysis of zou and iku2 mutants suggests that the final seed size may then be fine-tuned by the mechanosensitive regulation of genes such as ELA1 within this cell layer in response to pressure exerted by the zygotic compartment (our interpretation is presented schematically in Fig. 4e ). ELA1 and ELA2 are involved in the deactivation of bioactive GAs, potent stimulators of expansion which act, in part, by regulating the transcription of cell wall-modifying enzymes [23] , [24] , [26] . Until now, no direct link has been demonstrated between the regulation of GA levels and responses to mechanical stress. We propose that ELA1 may provide such a link. Plant growth conditions and transformation For staged materials, plants were grown under continuous light at 16 °C to slow down development, and flowers were emasculated and hand pollinated to ensure maximum synchronicity. Otherwise plants were grown under standard long-day conditions (21 °C, 16 h light/8 h dark). Comparisons were carried out on plants grown side by side under identical conditions. Agrobacterium -mediated plant transformation was carried out using the floral dip method [27] . In brief, the plants were allowed to bolt. Agrobacterium strains containing desired binary vectors were grown plated at high density onto YEB plates with the suitable antibiotics and incubated at 28 °C for 2–3 days. Bacteria were scraped off plates into 30 ml of LB to give an OD 600 of around 2.0. This solution was diluted in four volumes of a solution containing 5% sucrose and 0.03% Silwet L-77 (surfactant; Lehle Seeds). Plants were dipped in the solution for 10 s, with gentle agitation, covered with plastic bags for 24 h and then allowed to set seed. TEM analysis of cell wall structure Seeds for transmission electron microscopy analysis was removed from siliques by removal of the replum tissue with attached seeds, fixed in paraformaldehyde 3.2%+glutaraldehyde 2.5% in 0.1 M phosphate buffer (pH7.2) overnight at 4 °C, rinsed, postfixed in 1% OsO 4 in phosphate buffer overnight at 4 °C, rinsed, stained with tannic acid (1% in water) for 30 min, rinsed, dehydrated through an ethanol series and impregnated in increasing concentrations of SPURR [28] resin over a period of 4 days before being polymerized at 70 °C for 19 h, sectioned (65 nm sections) and imaged at 80 kV using an FEI TEM tecnai Spirit with 4 k × 4 k eagle ccd. Immunolocalization and calcofluor staining of seeds Seeds were fixed in ice-cold PEM buffer (50 mm PIPES, 5 mm EGTA and 5 mm MgSO 4 , pH 6.9) containing 4% (w/v) paraformaldehyde. Samples were placed under vacuum (3 × 30 min on ice), rinsed in PBS, dehydrated through an ethanol series and infiltrated with increasing concentrations of LR White resin in absolute ethanol (London Resin Company) over 8 days before being polymerized at 60 °C. Sections (1.0 μm) were cut using a glass knife on a Leica RM6626 microtome. Sections were incubated in PBS containing 3% (w/v) milk protein and a 10-fold dilution of antibody hybridoma supernatant (LM19, Plant Probes) [11] for 1 h, washed and incubated with a 100-fold dilution of fluorescently labelled (ab96963, Abcam) for 1 h in the dark. Samples were washed and counterstained with filtered Calcofluor White M2R (fluorescent brightener 28; Sigma-Aldrich) at 0.25 μg ml −1 and mounted in VECTASHIELD (Eurobio). Microscopy Living seeds were imaged by opening siliques on adhesive tape on the base of a small Petri dish, submerging in water and imaging using a dipping lens with a long working distance. When stated, seeds were stained by incubating for 10 min in 5 mg ml −1 propidium iodide, and rinsing twice before mounting in water. Confocal imaging was carried out on a Zeiss LSM700. Fluorescence and light microscopy imaging was carried out using a Zeiss axioimager 2. Molecular analysis Total RNA was extracted using the Spectrum Plant Total RNA Kit (Sigma). Total RNAs were digested with Turbo DNA-free DNase I (Ambion) according to the manufacturer’s instructions. RNA was reverse transcribed using the SuperScript VILO cDNA Synthesis Kit (Invitrogen) according to the manufacturer’s protocol. PCR reactions were performed in an optical 96-well plate in the StepOne Plus Real Time PCR System (Applied Biosystems), using FastStart Universal SYBR Green Master (Rox) (Roche), in a final volume of 20 μl, according to the manufacturer’s instructions. The following standard thermal profile was used for all PCR reactions: 95 °C for 10 min, 40 cycles of 95 °C for 10 s, and 60 °C for 30 s. Data were analysed using the StepOne Software v2.2 (Applied Biosystems). As a reference, primers for the EIF4A cDNA were used. PCR efficiency ( E ) was estimated from the data obtained from standard curve amplification using the equation E =10 −1/slope . Expression levels are presented as E −Δ C t , where Δ C t= C t GOI − C t EIF4A . Primers are listed in Supplementary Table 1 . The ELA1 promoter was amplified using primers listed in Supplementary Table 1 and cloned using restriction enzymes (BamH1 and Not1) into a modified version of pDONR P4-P1R (Life Technologies), before being incorporated into final constructions using Gateway technology. The ELA1/ELA2 amiRNA construct was designed using a web-based microRNA designer ( http://wmd3.weigelworld.org/cgi-bin/webapp.cgi ) and cloned into pDONR 221 (Life Technologies). Triple recombinations of appropriate entry vector combinations were performed into either pART27 (ref. 29 ; kanamycin resistance) or pH7m34GW [30] (hygromycin resistance). DNA templates for the probes used in in situ hybridizations were amplified using the primers listed in Supplementary Table 1 . Digoxigenin-labelled RNA probes were produced and hybridized to tissue sections following standard procedures. In brief, siliques were opened, fixed overnight in ice-cold PBS containing 4% paraformaldehyde, dehydrated through an ethanol series, embedded in Paraplast Plus (Mc Cormick Scientific) and sectioned (8 μm). Immobilized sections were dewaxed and hydrated, treated with 2 × saline sodium citrate (15 min), digested for 30 min at 37 °C with proteinase K (20 μg ml −1 in 50 mM Tris-HCl, pH 7.5, 5 mM EDTA), treated for 2 min with 0.2% glycine in PBS, rinsed, postfixed with 4% paraformaldehyde in PBS (10 min, 4 °C), rinsed, treated with 0.25% w/v acetic anhydride in 100 mM triethanolamine (pH 8.0 with HCl) for 10 min, rinsed and dehydrated. Sections were then hybridized under coverslips overnight at 50 °C with RNA probes (produced using DIG RNA labelling kit (Roche)) diluted in DIG easy Hyb solution (Roche) following the manufacturer’s instructions. Following hybridization, the slides were extensively washed in 0.1 × saline sodium citrate and 0.5% SDS at 50 °C (3 h), blocked for 45 min in 1% blocking solution (Roche) in TBS and for 45 minutes in BSA solution (1% BSA, 0.3% Triton-X-100, 100 mM Tris-HCl, 100 mM NaCl, 50 mM MgCl 2 ), and then incubated in a 1/1,000 dilution of in alkaline phosphatase-conjugated anti-digoxigenin antibody (Roche) in BSA solution for 2 h at RT. Sections were extensively washed in BSA solution, rinsed and treated overnight in the dark with a buffered NBT/BCIP solution. Samples were rinsed in water before air drying and mounting in Entellan (Sigma). Tissue compressions and microinjection experiments Microinjection experiments were carried out using an Eppendorf Femtojet microinjection and micromanipulation apparatus equipped with Femtotips II injecting needles (inner diameter 0.5 μm, outer diameter 0.7 μm). Seed compression experiments were performed using a custom tissue vice described in Supplementary Fig. 4 . Quantification of nuclear fluorescence was carried out using standard software in the ImageJ image analysis package [31] . Analysis of microtubule anisotropy was carried out using the ImageJ plug in FibrilTool [32] . How to cite this article: Creff, A. et al. A mechanically sensitive cell layer regulates the physical properties of the Arabidopsis seed coat. Nat. Commun. 6:6382 doi: 10.1038/ncomms7382 (2015).